Suppression of the critical thickness threshold for conductivity at the LaAlO3/SrTiO3interface Perovskite materials engineered in epitaxial heterostructures have been intensely investigated during the last decade. The interface formed by an LaAlO 3 thin film grown on top of a TiO 2 -terminated SrTiO 3 substrate hosts a two-dimensional electronic system and has become the prototypical example of this field. Although controversy exists regarding some of its physical properties and their precise origin, it is universally found that conductivity only appears beyond an LaAlO 3 thickness threshold of four unit cells. Here, we experimentally demonstrate that this critical thickness can be reduced to just one unit cell when a metallic film of cobalt is deposited on top of LaAlO 3 . First-principles calculations indicate that Co modifies the electrostatic boundary conditions and induces a charge transfer towards the Ti 3 d bands, supporting the electrostatic origin of the electronic system at the LaAlO 3 /SrTiO 3 interface. Our results expand the interest of this low-dimensional oxide system from in-plane to perpendicular transport and to the exploration of elastic and inelastic tunnel-type transport of (spin-polarized) carriers. Combined in heterostructures, oxide thin films offer a new playground with virtually unlimited combinations to realize artificial systems and to explore emerging phenomena absent in bulk compounds [1] . Ohtomo and Hwang [2] striking discovery of conducting LaAlO 3 /SrTiO 3 heterointerfaces has fast-tracked this system as the fruit fly for such investigations. The LaAlO 3 /SrTiO 3 system exhibits gate-tunable quasi-two-dimensional electronic conduction [3] , Rashba spin–orbit interaction [5] , [4] and superconductivity [6] , [7] , [8] , displays indications of magnetism [9] , [10] and even close coexistence of the latter two [11] , [12] , [13] . This makes the LaAlO 3 /SrTiO 3 system attractive for fundamental studies as well as promising for potential applications such as oxide-based electronics [14] , [15] , [16] . While the perovskite crystals LaAlO 3 (LAO) and SrTiO 3 (STO) are both wide band-gap insulators, the growth of an epitaxial LAO film on a TiO 2 -terminated, (001)-oriented STO substrate leads to an insulator-to-metal transition when the LAO thickness reaches 4 unit cells (uc) [3] . Owing to their ionic nature, the STO(001) substrate (non-polar) and the LAO(001) film (polar) form a strongly polar interface. This results in an electrostatic potential that increases as the LAO thickness is increased, leading to an electronic reconstruction with charge transferred towards the STO top-TiO 2 subplane [17] . Recently, first-principles calculations predicted a conductive system at the LAO/STO interface for heterostructures with various metallic capping layers, and an LAO thickness of 2 uc [18] . In this letter, we present results of electrical magnetotransport and X-ray absorption spectroscopy (XAS) experiments on LAO/STO samples with either bare LAO surfaces or a metallic capping layer of cobalt, combined with density functional theory (DFT) calculations. We demonstrate the existence of metallic conductivity on the STO side for an LAO thickness as thin as 1 uc. Magnetotransport measurements of Co/LAO/STO samples LAO films were grown by pulsed laser deposition (PLD) on TiO 2 -terminated STO(001) substrates and followed by in situ magnetron sputtering deposition of a 2–2.5-nm cobalt thin film, capped with a 3-nm AlO x layer to prevent Co oxidation. Details concerning samples fabrication and characterization can be found in the Methods section and in the Supplementary Information ( Supplementary Note 1 ). The unpatterned samples were electrically contacted with aluminium wires by ultrasonic wedge bonding. Four-point transport measurements (in-plane longitudinal R xx and transverse R xy magnetoresistances) were performed by connecting the corners of the square sample in the van der Pauw geometry. 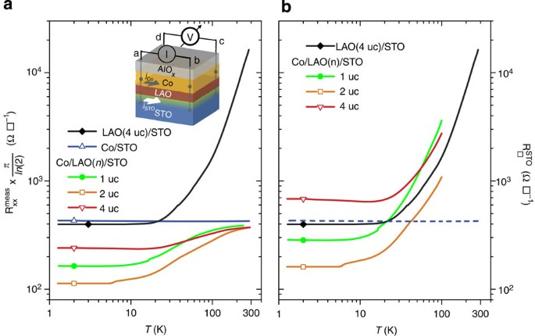Figure 1: Sheet resistances as a function of temperature. (a) Measured longitudinal resistanceRxxmeasversus temperatureTof LAO(4 uc)/STO and Co/LAO(n)/STO samples showing a clear metallic behaviour. The Co/STO resistance remains almost unchanged from 300 to 1.4 K (ΔR/R<1%). Inset: measurement configuration. The thick arrows in the sketch represent the current flowing in the Co layer and in the STO. (b) Calculated sheet resistanceof the conducting STO sublayer in Co/LAO(n)/STO samples (according to equation (1)), and measured sheet resistance of the LAO(4 uc)/STO samples. The blue dotted line corresponds to the Co/STO data set. Figure 1a shows the measured in-plane longitudinal resistance R xx meas versus temperature of Co/LAO/STO heterostructures with various LAO thicknesses, and of a Co/STO control sample for which the STO substrate experienced the same procedure of thermal and oxygen pressure cycles as for the LAO/STO samples. While the Co/STO sample shows very little variation of its resistance (<1%) across the explored temperature range, the Co-capped LAO/STO samples display a strong reduction in their resistance as temperature is decreased, which readily suggests that the LAO/STO interface conducts, even for samples with an LAO film thickness smaller than 4 uc. Figure 1: Sheet resistances as a function of temperature. ( a ) Measured longitudinal resistance R xx meas versus temperature T of LAO(4 uc)/STO and Co/LAO( n )/STO samples showing a clear metallic behaviour. The Co/STO resistance remains almost unchanged from 300 to 1.4 K (Δ R/R <1%). Inset: measurement configuration. The thick arrows in the sketch represent the current flowing in the Co layer and in the STO. ( b ) Calculated sheet resistance of the conducting STO sublayer in Co/LAO( n )/STO samples (according to equation (1)), and measured sheet resistance of the LAO(4 uc)/STO samples. The blue dotted line corresponds to the Co/STO data set. Full size image Following these observations, we now model the Co/LAO( n ≥1 uc)/STO heterostructures by two conducting layers in parallel composed of the Co overlayer and the STO sublayer. According to this simple picture, and supposing a temperature-independent resistance of the Co capping layer (see Fig. 1a ; Supplementary Fig. 1 ), the temperature evolution of the STO sublayer's longitudinal resistance is given by: The sheet resistance of the STO sublayer is defined as , assuming a homogeneous conductance in the geometry of the inset of Fig. 1a [19] , supported by the fact that R xx ≈ R yy within a few percent. For each sample, we calculate by taking the data set as , and as the measured value at room temperature ( ) for the corresponding sample. Figure 1b displays the calculated sheet resistance of the Co/LAO/STO samples in the low-temperature range (below 100 K). Next, we focus on transport experiments carried out in Hall configuration at room temperature and at low temperature (1.4 K). The measured transverse magnetoresistance curves were antisymmetrized ( ). Antisymmetrized traces R ac−db ( H ) and R db−ca ( H ) appear indistinguishable in Fig. 2a,b , suggesting again good sample homogeneity and no artefacts due to the data analysis. In the case of the LAO(4 uc)/STO sample, Hall measurements taken at room temperature show a linear behaviour for magnetic field up to 4 T (see Fig. 2a ) with an extracted sheet carrier densitiy n □ =6.4 × 10 13 cm −2 . In contrast, Co/STO and Co/LAO/STO samples exhibit at room temperature a Hall effect dominated by the cobalt layer, independent of the LAO thickness (see inset of Fig. 2a ), with a low-magnetic-field regime (| μ 0 H |≤1.2 T) displaying the anomalous Hall effect characteristic of a ferromagnetic metal. In the high-field regime (| μ 0 H |≥2.2 T), the Co magnetization is rotated out of plane and the Co-capped samples exhibit a normal Hall effect with a weak negative slope of order −10 mΩ T −1 (that is a carrier density of order 10 23 cm −3 ). 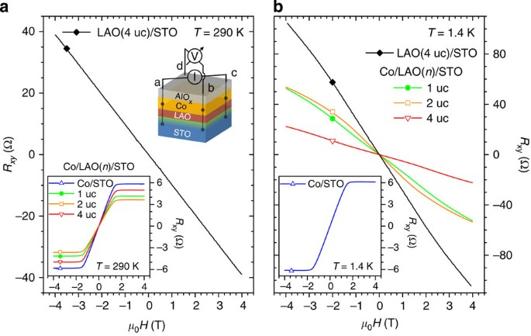Figure 2: Hall effect measurements. (a) Antisymmetrized Hall resistanceRxyas a function of applied magnetic fieldμ0Hof an LAO(4 uc)/STO sample displaying a linear Hall effect at room temperature. Inset:Rxyversusμ0Hfor various Co/LAO(n)/STO samples at 290 K showing cobalt dominated AHE at low magnetic field. (b) Antisymmetrized Hall resistanceRxyversusμ0Hof an LAO(4 uc)/STO sample and of Co/LAO(n)/STO at 1.4 K. Inset:Rxyversusμ0Hfor Co/STO at 1.4 K similar to the one observed at 290 K. Figure 2: Hall effect measurements. ( a ) Antisymmetrized Hall resistance R xy as a function of applied magnetic field μ 0 H of an LAO(4 uc)/STO sample displaying a linear Hall effect at room temperature. Inset: R xy versus μ 0 H for various Co/LAO( n )/STO samples at 290 K showing cobalt dominated AHE at low magnetic field. ( b ) Antisymmetrized Hall resistance R xy versus μ 0 H of an LAO(4 uc)/STO sample and of Co/LAO( n )/STO at 1.4 K. Inset: R xy versus μ 0 H for Co/STO at 1.4 K similar to the one observed at 290 K. Full size image Figure 2b displays Hall data acquired at 1.4 K. R xy ( H ) measured at 1.4 K in Co/STO shows essentially no change when compared with room temperature measurements (see insets of Fig. 2a,b ). On the other hand, R xy ( H ) behaviour of Co/LAO( n =1,2,4 uc)/STO samples at 1.4 K display striking similarities with those carried out on uncapped LAO(4 uc)/STO samples. The Hall resistance trace of the LAO(4 uc)/STO sample is not purely linear at 1.4 K, a behaviour believed to arise from the multi-band structure of STO [20] , [21] , [22] . Evidence for this is given from the DFT calculations in the Supplementary Information (see Supplementary Fig. 2 ). We only consider the ‘high field’ regime (| μ 0 H |≥3 T) where n □ , the total electron density in the STO, is given by , with e the elementary charge and R H the Hall coefficient determined for | μ 0 H |≥3 T. The kink observed in the LAO(4 uc)/STO Hall trace R xy ( H ) is well reproduced in Co-capped LAO samples at 1.4 K, regardless of the LAO thickness. This close resemblance for both sets of samples suggests a common host for the observed electronic transport. The measured Hall coefficients, and related carrier densities show no correlation with LAO thickness. Taking the sheet resistance and Hall coefficient at 1.4 K, one can estimate the electronic mobility of the STO sublayer in Co/LAO/STO samples. Values in the range of (1−6 × 10 2 cm 2 V −1 s −1 ) are found. We note that the very thin Co layer is not expected to play a role in Hall effect measurements at 1.4 K, owing to its much lower mobility ( <1 cm 2 V −1 s −1 determined experimentally), thus supporting our simple analysis. Hence, our transport data collected on Co/LAO/STO heterostructures clearly indicate the presence of an electronic system at the LAO/STO interface whose behaviour is very similar to the usual LAO( n ≥4 uc)/STO, even for LAO as thin as a single unit cell. Furthermore, the estimated carrier densities (several 10 13 – × 10 14 cm −2 ) in Co/LAO/STO samples are comparable to values typically found for quasi-two-dimensional electronic systems at LAO/STO interfaces [3] , [23] , [24] . X-ray absorption spectroscopy experiments To gain further insight into the electronic structure of Co/LAO/STO systems, we have performed XAS measurements at the DEIMOS beamline of Synchrotron SOLEIL [25] . XAS probes transition from core electronic states to excited electronic states. The energy of the incident X-ray beam can be tuned to the Ti L 2,3 absorption edge to probe electronic transitions from 2 p 3/2 and 2 p 1/2 to 3 d levels (see Fig. 3a ) [26] . Therefore, the preferential occupancy of states with different orbital symmetries can be probed by X-ray linear dichroism (XLD), which is the difference in XAS measured with a linear horizontal (LH) or vertical (LV) polarization of the X-ray beam (see Fig. 3b ], that is, XLD=(LH−LV). Conversely, the isotropic signal is defined as the mean of the two: ISO=(LH+LV)/2. 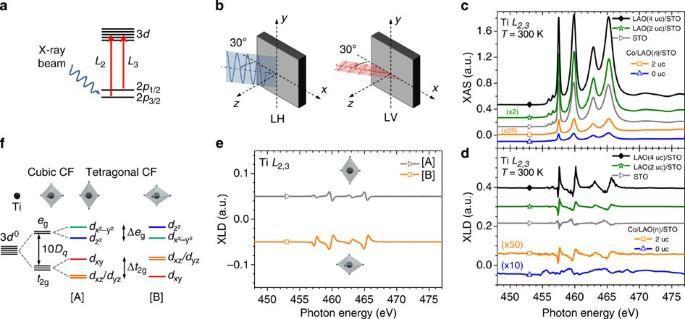Figure 3: X-ray absorption spectroscopy at TiLedge. (a) Sketch of the X-ray absorption spectroscopy (XAS) process depicting the 2p→3delectronic transitions at the TiL2,3edge. (b) Scheme of the XAS measurement geometries with linearly horizontal (LH) and linearly vertical (LV) polarized light. The incident beam forms a 30° angle with the sample surface (x,y). (c) Experimentally measured isotropic signals (ISO) versus photon energy of a STO(001) substrate, and of various (Co/)LAO(n)/STO samples. Spectra acquired at 300 K in total electron yield mode. (d) The corresponding experimental X-ray linear dichroism (XLD) signals show a sign inversion between the XLD of STO and Co/STO and that of LAO(2,4 uc) and Co/LAO(2 uc) samples. (e) Calculated XLD that reproduces the experimental XLD of the STO bare substrate (circle, [A]) and of the Co/LAO(2 uc)/STO sample (square, [B]). (f) The cubic crystal field (CF) splits the Ti4+3dstates intoegandt2glevels. A tetragonal CF further lifts the orbital degeneracy, with: [A] case of STO, [B] case of (Co/)LAO/STO. Figure 3: X-ray absorption spectroscopy at Ti L edge. ( a ) Sketch of the X-ray absorption spectroscopy (XAS) process depicting the 2 p →3 d electronic transitions at the Ti L 2,3 edge. ( b ) Scheme of the XAS measurement geometries with linearly horizontal (LH) and linearly vertical (LV) polarized light. The incident beam forms a 30° angle with the sample surface (x,y). ( c ) Experimentally measured isotropic signals (ISO) versus photon energy of a STO(001) substrate, and of various (Co/)LAO( n )/STO samples. Spectra acquired at 300 K in total electron yield mode. ( d ) The corresponding experimental X-ray linear dichroism (XLD) signals show a sign inversion between the XLD of STO and Co/STO and that of LAO(2,4 uc) and Co/LAO(2 uc) samples. ( e ) Calculated XLD that reproduces the experimental XLD of the STO bare substrate (circle, [A]) and of the Co/LAO(2 uc)/STO sample (square, [B]). ( f ) The cubic crystal field (CF) splits the Ti 4+ 3 d states into e g and t 2g levels. A tetragonal CF further lifts the orbital degeneracy, with: [A] case of STO, [B] case of (Co/)LAO/STO. Full size image The XAS experiments were performed at the Ti L 2,3 absorption edge, on the same Co/STO and Co/LAO(2 uc)/STO samples previously shown in Figs 1 and 2 , as well as on a bare STO substrate, on an insulating LAO(2 uc)/STO heterostructure and on a conducting LAO(4 uc)/STO sample. All spectra were collected at 300 K in total electron yield mode in order to be surface sensitive. In Fig. 3 , the ISO signals appear to be largely of Ti 4+ character for all samples [27] . The XLD signals, however, display significant differences between the samples (see Fig. 3d ). In LAO/STO samples with 2 and 4 uc of LAO, the XLD shows a sign reversal with respect to that obtained from a bare STO substrate. This is related to an inverted (negative versus positive) splitting of the 3 d bands (see Fig. 3f ). Interestingly, the XLD measured on the Co/LAO(2 uc)/STO sample is also very different from that of the STO substrate and appears very similar to the uncapped LAO/STO samples. Although much noisier, the XLD signal of the Co/STO sample resembles that of the bare STO. In bulk cubic STO, the crystal field splits the fivefold degenerate Ti 3 d bands into twofold and threefold t 2g ( d xy , d xz , d yz ) degenerate bands [28] . In an attempt to clarify this band picture, we have performed atomic multiplet calculations using the CTM4XAS program [29] . It allowed us to explore the effect of a symmetry reduction of the system (for example, towards tetragonal), which distorts the TiO 6 octahedra and lifts the degeneracy of the e g and t 2g bands (see Fig. 3e,f ). The measured XLD were well reproduced by using values of the energy splittings identical to those reported in the literature [30] , [31] . In the case of STO, we considered positive energy splittings Δ e g =40 meV and Δ t 2g =25 meV [30] . In contrast, for the LAO/STO and Co/LAO/STO systems, negative energy splittings Δ e g =−100 meV and Δ t 2g =−50 meV were considered [31] . We note that introducing a Co capping layer does not alter the fine structure of the XLD observed in uncovered LAO/STO samples. Interestingly, we have shown that Co-capped and uncapped LAO/STO systems have a similar subband structure, with a preferential d xy orbital occupancy. Incidentally, we performed X-ray magnetic circular dichroism experiments at the Ti L 2,3 edge on Co/LAO( n )/STO samples with n =2 and 4 uc samples (see Supplementary Fig. 3 ). The signal-to-noise ratio of our experiments allows us to estimate the Ti magnetic moment averaged over the total probing depth to be of the order of 10 −2 μ B per atom ( Supplementary Note 2 ). This value is in agreement with those obtained from the DFT calculations presented below as well as from neutron reflectometry on LAO/STO superlattices [32] and recent X-ray magnetic circular dichroism experiments on similarly prepared LAO/STO-conducting interfaces [33] . First-principles calculations To elucidate the origin of the observed onset of conductivity below 4 uc of LAO, DFT calculations were performed on Co( m )/LAO( n )/STO(001) (see Fig. 4 ) with the all-electron full-potential linearized augmented plane wave, as implemented in the WIEN2k code [34] , [35] . For the exchange-correlation functional, we used the generalized gradient approximation (GGA) [36] . The influence of electronic correlations beyond GGA is discussed in the Supplementary Note 3 (see also Supplementary Fig. 4 ). The in-plane lattice parameter is set to the GGA equilibrium lattice constant of STO ( a STO =3.92 Å) and the atomic positions are fully relaxed within tetragonal symmetry. More details are provided in ref. 18 (see also the Methods section and Supplementary Note 3 ). 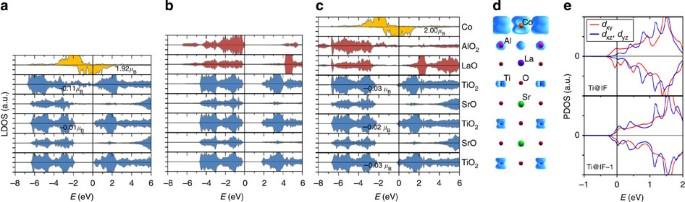Figure 4: Layer-resolved density of states. LDOS of (a) Co(1 ML)/STO, (b) LAO(1 uc)/STO and (c) Co(1 ML)/LAO(1 uc)/STO heterostructures within GGA with a 4.5-uc-thick STO substrate. (d) Side view of Co(1 ML)/LAO(1 uc)/STO with the electron density integrated in the intervalEF−0.50 eV toEF, giving insight into the Ti 3dorbital occupation, where corresponds to the Fermi level. (e) Projected density of states (PDOS) of Ti in the interface (IF) and IF-1 layer of Co/LAO(1 uc)/STO. Positive (negative) values correspond to majority (minority) spin. Figure 4a shows the layer-resolved density of states of a (001)-oriented STO substrate (4.5-uc thick) covered with one monolayer (ML) of Co. In contrast to the uncovered STO(001) substrate (not shown here), where the Fermi level is pinned at the top of the valence band defined by surface states at the topmost TiO 2 layer, for Co/STO(001) the Fermi energy E F shifts to the bottom of the Ti conduction band, leaving the Ti 3 d band empty. Figure 4: Layer-resolved density of states. LDOS of ( a ) Co(1 ML)/STO, ( b ) LAO(1 uc)/STO and ( c ) Co(1 ML)/LAO(1 uc)/STO heterostructures within GGA with a 4.5-uc-thick STO substrate. ( d ) Side view of Co(1 ML)/LAO(1 uc)/STO with the electron density integrated in the interval E F −0.50 eV to E F , giving insight into the Ti 3 d orbital occupation, where corresponds to the Fermi level. ( e ) Projected density of states (PDOS) of Ti in the interface (IF) and IF-1 layer of Co/LAO(1 uc)/STO. Positive (negative) values correspond to majority (minority) spin. Full size image A similar change is observed when capping LAO/STO(001) with Co: In the uncovered LAO(1 uc)/STO system, the Fermi level lies at the top of the valence band (see Fig. 4b ), determined by O 2 p states of the surface AlO 2 layer, while the conduction band minimum is 2 eV above the Fermi energy and is determined by Ti 3 d states. Adding a Co capping layer shifts the Fermi level to the bottom of the conduction band in Co/LAO(1 uc)/STO (see Fig. 4c ). In contrast to LAO(1 uc)/STO and Co/STO, in Co/LAO(1 uc)/STO the Ti 3 d band is now partially occupied, with a small spin polarization of −0.02 to −0.03μ B per Ti. Hence a metallic bilayer is formed in Co/LAO/STO, with a conducting surface (Co) and a conducting burried interface (STO side), consistent with the transport data. Furthermore, the Ti 3 d band occupation increases weakly with LAO thickness (see Supplementary Figs 5 and 6 ). Adding the Co capping layer (largely) cancels the internal potential buildup within the polar LAO film. As found previously [18] , the position of the Fermi level with respect to the conduction band minimum in STO is determined by the work function of the metallic contact (4.72 eV for 1 ML Co and 4.28 eV for 3 ML Co). This, together with the still persisting polar discontinuity at the LAO/STO interface leads to a finite occupation of the Ti 3 d band at the interface. Next, we explore the preferential orbital occupancy of the electronic system. The electron density of Co/LAO(1 uc)/STO, integrated between E F −0.50 eV and E F reveals predominant d xy orbital polarization of Ti in the interface layer and d xz / d yz character in deeper layers (see Fig. 4d ), which can also be seen on the projected density of states in Fig. 4e . The orbital polarization is consistent with the structural distortions of the octahedra within the Co/LAO(1 uc)/STO heterostructure: We find that the average distance between the apical oxygens on both sides of Ti in the [001] direction is 3.92 Å for the interfacial (IF) and 3.99 Å for the IF-1 layers, respectively. In line with the experimentally determined t 2g splittings ( Fig. 3d–f ), we find that a shortened (expanded) TiO 6 octahedra average size in the [001] direction corresponds to d xy orbitals lying lower (higher) in energy. Using four-point transport experiments, we have revealed the presence of metallic conduction at the LaAlO 3 /SrTiO 3 interface for Co/LaAlO 3 ( n )/SrTiO 3 heterostructures with LaAlO 3 thicknesses 1 uc≤ n ≤4 uc. The linear dichroism observed through XAS evidences a compressive tetragonal distortion of the TiO 6 octahedra for cobalt-capped and uncapped LaAlO 3 /SrTiO 3 systems. Making use of atomic multiplet calculations, we found that in Co/LaAlO 3 /SrTiO 3 the Ti orbitals reconstruct from the situation in bare SrTiO 3 substrates. As a result, the lowest energy level has a d xy orbital character for Co/LaAlO 3 /SrTiO 3 systems, compared with d xz / d yz for the bare SrTiO 3 . DFT calculations support this picture and predict structural distortions that agree with those inferred from XAS. Further, they indicate a finite occupancy of the Ti 3d bands at the Fermi energy for the Co/LaAlO 3 (1 uc)/SrTiO 3 heterostructure, with a predominant d xy orbital character within the interfacial TiO 2 layer. The metallic Co overlayer thus appears to modify the electrostatic boundary conditions of the LAO/STO system, leading to the occupation of the Ti 3 d bands. These observations support the electrostatic origin of the quasi-two-dimensional electronic systems at the LAO/STO interface as proposed in the polar catastrophe model [17] , [37] , which suggests that cationic intermixing across the interface [38] or oxygen vacancies [39] , [40] , [41] only play a marginal role. For spintronics and tunnelling spectroscopy applications, it is necessary to control the tunnel barrier resistance, which is usually achieved by tuning its thickness. In the LaAlO 3 /SrTiO 3 case, a stringent limitation for efficient tunnelling was the existence of a minimum thickness of 4 uc of LaAlO 3 for the onset of conductivity. Our findings should therefore considerably facilitate spin injection [42] , [43] or tunnel spectroscopy studies [44] , [45] , [46] only achievable in perpendicular geometries, thereby paving the way toward LaAlO 3 /SrTiO 3 -based electronic and spintronic tunnelling devices with tunable tunnel resistances. Samples fabrication The LaAlO 3 (LAO) films were grown by PLD on 5 × 5 mm TiO 2 -terminated (001)-oriented SrTiO 3 (STO) substrates. A single-crystal LAO target was ablated by a KrF (248 nm) excimer laser at a repetition rate of 1 Hz and with a fluence of ~\n1 J cm −2 . The LAO deposition was performed in an oxygen partial pressure of 2.0 × 10 −4 mbar and at a substrate temperature of 730°C. Substrate-to-target distance was 63 mm. The layer-by-layer growth mode allowed us to precisely control the LAO thickness through real-time monitoring of reflection high-energy electron diffraction intensity oscillations (see Fig. 5a ). The samples were then annealed for 30 min in about 400 mbar of oxygen at 500°C (refs 39 , 40 ). Finally, the LAO/STO heterostructures were cooled at 25 °C min −1 and kept in the same oxygen pressure for ~\n30 to 60 min. PLD growth was followed by in situ deposition of a metallic cobalt electrode by magnetron sputtering at room temperature in a pure Ar atmosphere of 4.5 × 10 −4 mbar, resulting in a clean Co/LAO interface. The 2–2.5-nm Co thin films were capped with a 3-nm AlO x layer to prevent cobalt oxidation. For the Co/STO sample, the same procedure of thermal and pressure cycles as the one described above were applied to the TiO 2 -terminated STO substrate, skipping only the LAO deposition step, before the Co deposition. 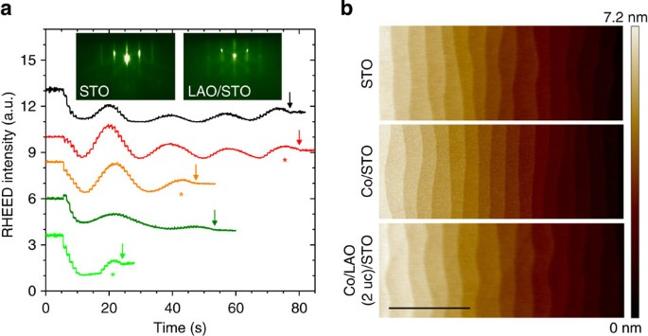Figure 5:In situRHEED andex situAFM characterizations. (a) Monitoring of the RHEED (01) diffraction peak intensity versus time during the epitaxial growth of LAO films of various thicknesses (1–4 uc) on STO substrates. Inset: typical RHEED pattern of (left) an STO substrate, and (right) a 4-uc LAO thin film on STO, taken at 730°C in an oxygen partial pressure of 2.0 × 10−4mbar. Arrows indicate the end of the growth. Asterisks designate samples later covered with a Co/AlOxcapping. (b) AFM topography of a TiO2-terminated STO substrate and of Co/STO and Co/LAO(2 uc)/STO samples. The 2-nm Co thin film reproduces the steps and terraces of the terminated substrate. Scale bar, 1 μm. Figure 5: In situ RHEED and ex situ AFM characterizations. ( a ) Monitoring of the RHEED (01) diffraction peak intensity versus time during the epitaxial growth of LAO films of various thicknesses (1–4 uc) on STO substrates. Inset: typical RHEED pattern of (left) an STO substrate, and (right) a 4-uc LAO thin film on STO, taken at 730°C in an oxygen partial pressure of 2.0 × 10 −4 mbar. Arrows indicate the end of the growth. Asterisks designate samples later covered with a Co/AlO x capping. ( b ) AFM topography of a TiO 2 -terminated STO substrate and of Co/STO and Co/LAO(2 uc)/STO samples. The 2-nm Co thin film reproduces the steps and terraces of the terminated substrate. Scale bar, 1 μm. Full size image AFM characterization We performed an atomic force microscopy (AFM) topography study of uncapped 2-nm Co films grown on a TiO 2 -terminated STO substrate and on an LAO/STO sample (see Fig. 5b ). The Co was left to oxidize in air, which we believe could only increase surface roughness compared with Co metallic films capped with AlO x . We estimate the root mean square surface roughness value ( R q ) of the Co film by averaging over four 3 × 3 μm 2 images from different locations across the sample. R q =1.49 Å and 1.33 Å for Co films grown on the STO substrate and the LAO(2 uc)/STO, respectively. For comparison, the surface roughness of a terminated STO substrate from the same batch is of 1.50 Å. The surface roughness values are in fact dominated by the vicinal atomic steps and terraces of the substrate: considering 3.9 Å steps height leads to R q =1.13 Å. The AFM characterization study supports the smoothness and continuity of the 2-nm Co layer and suggests full coverage of the STO or LAO surfaces by the Co thin films. DFT calculations DFT calculations were performed using the all-electron full-potential linearized augmented plane wave method, as implemented in the WIEN2k code [34] , [35] . For the exchange-correlation potential, we used the GGA [36] . The muffin-tin spheres of the atoms were taken as: 2.3, 1.8 and 1.6 a.u. for La/Sr, Ti/Co/Al and O, respectively. The energy cutoff for the plane wave representation in the interstitial is for the wave functions. The spherical harmonics inside the muffin-tin spheres are expanded up to l max =10, while the plane wave expansion of the charge density was truncated at G max =12 a.u. −1 , where a.u. stands for atomic units.. The integrals over the Brillouin zone are performed with 36 k -points in the irreducible part of the Brillouin zone using the Monkhorst-Pack special k -points approach [47] . We have chosen a symmetric slab with LAO and Co layers on both sides of the 4.5-uc-thick STO substrate and a vacuum region between the slab and its periodic images of at least 10 Å. The Co atoms are adsorbed on top of the oxygen ions at the surface of TiO 2 or AlO 2 . The in-plane lattice parameter is set to the GGA equilibrium lattice constant of STO ( a STO =3.92 Å), and the atomic positions are fully relaxed within tetragonal symmetry. How to cite this article: Lesne, E. et al . Suppression of the critical thickness threshold for conductivity at the LaAlO 3 /SrTiO 3 interface. Nat. Commun. 5:4291 doi: 10.1038/ncomms5291 (2014).